Modification of the carboxy-terminal flanking region of a universal influenza epitope alters CD4+T-cell repertoire selection Human CD4 + αβ T cells are activated via T-cell receptor recognition of peptide epitopes presented by major histocompatibility complex (MHC) class II (MHC-II). The open ends of the MHC-II binding groove allow peptide epitopes to extend beyond a central nonamer core region at both the amino- and carboxy-terminus. We have previously found that these non-bound C-terminal residues can alter T cell activation in an MHC allele-transcending fashion, although the mechanism for this effect remained unclear. Here we show that modification of the C-terminal peptide-flanking region of an influenza hemagglutinin (HA 305−320 ) epitope can alter T-cell receptor binding affinity, T-cell activation and repertoire selection of influenza-specific CD4 + T cells expanded from peripheral blood. These data provide the first demonstration that changes in the C-terminus of the peptide-flanking region can substantially alter T-cell receptor binding affinity, and indicate a mechanism through which peptide flanking residues could influence repertoire selection. Defence against invading pathogens is the primary function of the immune system. To this end, jawed vertebrates have evolved an elaborate recombinatorial system to generate a hugely diverse range of cell surface-expressed antigen receptors that enable the selection and expansion of pathogen-specific cell populations in response to infection. Heterodimeric αβ T-cell receptor (TCR) binding to cognate peptide-major histocompatibility complex (pMHC) antigen underpins the effective activation of specific T-cell populations [1] . These primary recognition events occur in the context of a naïve T-cell pool that comprises ∼ 25×10 6 distinct TCR clonotypes [2] . TCR diversity is generated during the somatic rearrangement of T receptor ( TR ) genes and is driven mechanistically by the imprecise stochastic recombination of variable (V), diversity (D) and joining (J) gene segments, exonucleolytic activity, random non-templated nucleotide additions and differential chain pairing. The highly variable complementarity-determining region 3 (CDR3) is formed by the resulting VDJ segment for TCRβ chains; an analogous VJ recombination process generates CDR3α (ref. 3 ). Multiple TCR clonotypes can respond to an antigenic stimulus, and measurement of either CDR3β lengths or sequences within defined T-cell populations can provide an indication of repertoire size and variability [4] , [5] . CD4 + T cells recognize antigens presented by classical MHC-II molecules. Limited structural studies of TCR binding to pMHC-II have demonstrated that the CDR3 loops contact exposed residues in the epitope backbone and engender TCR specificity [6] . This docking strategy is akin to that observed within the more extensive structural dataset available for TCR binding to pMHC-I (ref. 6 ). In humans, the most frequent MHC-II presenting element is the human leukocyte antigen (HLA)-DR αβ heterodimer. The HLA-DR α-chain is monomorphic, whereas the β-chain is highly polymorphic and generates a binding motif for selected peptide epitopes [7] , [8] . The core epitope is a nonamer peptide bound through a series of pockets in the HLA-DR heterodimer at position (P)1, P4, P6 and P9. However, the binding groove of the HLA-DR heterodimer is open at either end, which allows longer peptides to bind with the non-bound flanking regions extending from the amino-terminus (for example, P − 1, P − 2) and carboxy-terminus (for example, P10, P11) of the peptide [9] . We have previously eluted and sequenced multiple ligands from a range of MHC-II molecules and identified not only core MHC-specific binding motifs, but also enrichment in the non-bound flanking residues, particularly basic residues at the C-terminus; this latter observation is allele-transcending [10] , [11] . Furthermore, it has been shown that residue alteration in the flanking regions of peptides can alter their immunogenicity, although the mechanism that underpins this observation is unknown [11] , [12] , [13] , [14] , [15] . Biophysical investigations of the TCR/pMHC interaction show that TCRs bind very weakly, compared for instance to antibodies, with equilibrium binding constants ( K D s) usually in the region of ∼ 10–100 μM; the strength and/or duration of the TCR/pMHC interaction are probably the chief parameters that govern T-cell activation [16] , [17] . By studying multiple TCR/pMHC interactions, we have found that pMHC-I-restricted TCRs bind with markedly stronger affinities (mean K D =13 μM) compared with pMHC-II-restricted TCRs (mean K D =52 μM) [18] . Although it is clear that there is a natural range of affinities within which a TCR functions, we have also found that the progression from agonist to weak agonist to antagonist peptide ligands reflects a steady decline in TCR/pMHC affinity [19] . Conversely, although augmented T-cell effector function might follow an increase in TCR/pMHC affinity, very high affinity interactions raise the possibility of cross-reactivity at the expense of specificity. The generation of effective CD4 + T-cell responses is critically important for protective immunity, both during infection and following vaccination. Indeed, even a transient failure of the CD4 + T-cell response may offer a window for pathogen persistence [20] . Primary T-cell responses are frequently broad and include low-avidity clonotypes owing to the efficiency of cognate naïve T-cell recruitment [21] , but the evolution of an effective T-cell response can involve preferential selection for fewer clonotypes with higher avidity interactions [22] , [23] , [24] . Strategies that augment or select a repertoire that comprises clonotypes with higher affinity TCRs may therefore be attractive from an interventional perspective, especially if this can be implemented without sacrificing antigen specificity. In this regard, substitutions of amino acids in the core epitope may be risky, because they can both alter TCR specificity and unpredictably affect TCR binding strength and subsequent T-cell activation [25] , [26] . Here we examine how substitutions in the non-core C-terminal flanking region of the well-characterized universal influenza hemagglutinin (HA 305−320 ) epitope [27] affect T-cell recognition and TCR selection. Multiple different amino-acid substitutions of residues in the C-terminus at P10 and P11 were tested against cognate T-cell clones. The effects of favourable substitutions on recognition by polyclonal cognate T cells derived from the memory pool were then explored, and biophysical analyses of TCR/pMHC-II binding were conducted using surface plasmon resonance (SPR) to provide molecular insight into these effects. These data provide the first demonstration that modifications to the C-terminal peptide-flanking region can directly alter TCR binding affinity and T-cell repertoire selection. Flu-specific CD4 + T cells prefer C-terminal basic residues Three CD4 + T-cell clones (HA-C6, HA-C5 and HA-CA), each specific for HLA-DR1/HA 305−320 (Flu1), were screened using IFN-γ ELISpot assays for recognition of peptides with a conserved core epitope (HA 309−317 ) but variant C-terminal flanking regions at either P10 (HA 318 ) or P11 (HA 319 ). A total of 22 different 16mer peptide variants of HA 305−320 , listed in the Methods, were tested in these assays. 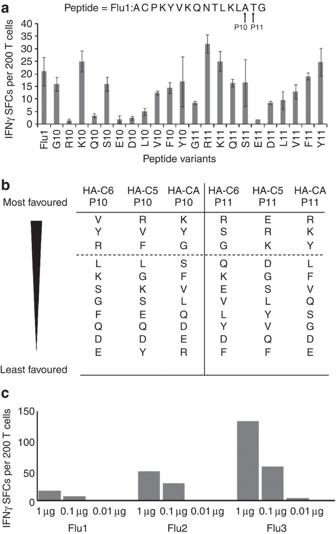Figure 1: Screening of Flu1-specific CD4+T-cell clones with peptide libraries. (a) Representative data generated by screening clone HA-CA with 22 flanking variant peptides using IFN-γ ELISpot assays to examine the effects of amino-acid substitutions at P10 or P11. Error bars shown are standard deviation from three separate experiments. (b) Summary of screening data generated with three different Flu1-specific CD4+T-cell clones (HA-C6, HA-C5 and HA-CA). Overall, the most favoured consensus alterations include basic residues at P10 and P11. (c) The Flu1-specific clone HA1.7 was stimulated with the indicated concentrations of the Flu1 peptide, or altered peptides with Arg at P10 (Flu2) or P11 (Flu3), in IFN-γ ELISpot assays. Representative data generated with the HA-CA clone are shown in Figure 1a . The most favoured to the least favoured substitutions were ranked for each clone ( Fig. 1b ), demonstrating a preference for positively charged basic residues (Lys, Arg) at P10 and P11. Indeed, a comparison across all three clones of basic/acidic residues versus all other amino acids in the top three recognition positions ( Fig. 1b ) revealed a significant enrichment of positively charged over negatively charged residues (Fisher's exact test P =0.0045). This striking reluctance to accept acidic residues is illustrated in the screening data generated with clone HA-CA, which showed reduced activation with Asp or Glu at either P10 or P11 ( Fig. 1a ). Although this particular clone did not favour Arg at P10, other clones showed a striking increase in responsiveness to altered peptides with an Arg at either P10 (Flu2) or P11 (Flu3) ( Fig. 1c ). Figure 1: Screening of Flu1-specific CD4 + T-cell clones with peptide libraries. ( a ) Representative data generated by screening clone HA-CA with 22 flanking variant peptides using IFN-γ ELISpot assays to examine the effects of amino-acid substitutions at P10 or P11. Error bars shown are standard deviation from three separate experiments. ( b ) Summary of screening data generated with three different Flu1-specific CD4 + T-cell clones (HA-C6, HA-C5 and HA-CA). Overall, the most favoured consensus alterations include basic residues at P10 and P11. ( c ) The Flu1-specific clone HA1.7 was stimulated with the indicated concentrations of the Flu1 peptide, or altered peptides with Arg at P10 (Flu2) or P11 (Flu3), in IFN-γ ELISpot assays. Full size image CD4 + T-cell clonotypic responses to modified Flu-epitopes Peptides modified in their non-core bound C-terminal flanking region seemed to alter the degree of T-cell activation. To examine this observation further, we used modified peptides to expand CD4 + T cells from the influenza-specific memory pool of two HLA-DR1 + donors (known responders to HA 305−320 ). Ten-day cultures of 10 6 peripheral blood mononuclear cells (PBMCs) with the peptides Flu1 (wild-type sequence) or Flu2 (Arg at P10) expanded ≥5×10 4 CD4 + HLA-DR1/HA 305−320 tetramer-positive cells (data not shown). We investigated TCR usage by these amplified populations (Flu1 versus Flu2) to establish whether different repertoires were deployed against peptide epitopes with C-terminal modifications. Initially, we employed TCR spectratyping on HLA-DR1/HA 305−320 tetramer-sorted cells, comparing the immunoscope profiles of each T-cell receptor beta variable (TRBV) family the relative representation of each TRBV family in background peripheral blood, CD4 + T-cell lines expanded with the wild-type Flu1 peptide and, CD4 + T-cell lines expanded with the basic tail Flu2 peptide ( Fig. 2 ). 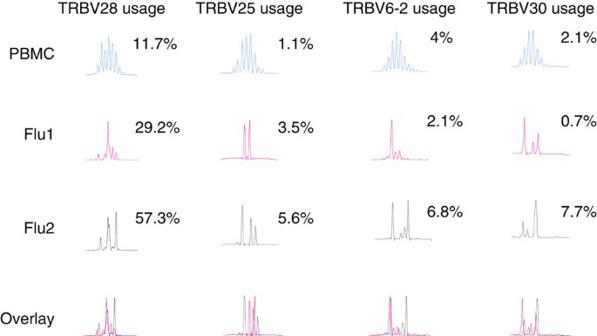Figure 2: Immunoscope profiles from CD4+T-cell lines expanded with Flu1 or Flu2 (Arg at P10). Short-term T-cell lines were generated from peripheral blood stimulated with either Flu1 or Flu2. Antigen-specific CD4+cells were isolated on the basis of HLA-DR1/HA305−320tetramer staining, and TCR repertoires were assessed by spectratyping. The profiles of pooled CDR3β lengths for four TRBV families are shown. In peripheral blood, the expected Gaussian distribution is observed. Altered profiles for the Flu1-specific and Flu2-specific populations indicate oligoclonal expansions. Differences in TRBV family usage are also apparent, suggesting that particular clonotypic expansions can be driven by a C-terminally modified peptide. A representative example from three independent experiments is shown. Figure 2: Immunoscope profiles from CD4 + T-cell lines expanded with Flu1 or Flu2 (Arg at P10). Short-term T-cell lines were generated from peripheral blood stimulated with either Flu1 or Flu2. Antigen-specific CD4 + cells were isolated on the basis of HLA-DR1/HA 305−320 tetramer staining, and TCR repertoires were assessed by spectratyping. The profiles of pooled CDR3β lengths for four TRBV families are shown. In peripheral blood, the expected Gaussian distribution is observed. Altered profiles for the Flu1-specific and Flu2-specific populations indicate oligoclonal expansions. Differences in TRBV family usage are also apparent, suggesting that particular clonotypic expansions can be driven by a C-terminally modified peptide. A representative example from three independent experiments is shown. Full size image The baseline range and polyclonality of the TCR repertoire was demonstrated in peripheral blood using specific primers to amplify each TRBV family and by analysing CDR3β length profiles within each TRBV family; for the latter, the expected Gaussian distribution pattern was observed ( Supplementary Fig. S1 ). Expansion of antigen-specific CD4 + T cells by peptide stimulation (Flu1 or Flu2) was reflected by distinct peaks in the immunoscope profiles, corresponding to individual T-cell clonotypes. The introduction of a C-terminal Arg at P10 in Flu2 led to both skewing of TRBV family usage and altered TCR representation within the expanded TRBV families ( Fig. 2 ). This experiment was repeated with another HLA-DR1 + donor; similar selective expansions within the CD4 + T-cell populations specific for Flu1 and Flu2 were observed (data not shown). The spectratyping analyses suggested that markedly altered expansions of memory T cells could be driven by the presence of Arg in the C-terminal non-core epitope flanking region. To dissect this repertoire disparity in more detail, we employed an unbiased template-switch anchored RT–PCR to characterize all expressed TRB gene products from tetramer-sorted CD4 + T-cell lines primed with wild-type, P10 or P11 Arg-substituted HA 305−320 peptides (Flu1, Flu2 and Flu3, respectively). 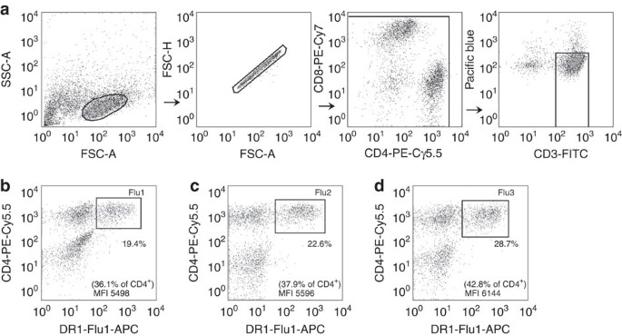Figure 3: Flow cytometric sorting of CD4+T-cell lines. Short-term T-cell lines were generated from peripheral blood stimulated with the indicated peptides. Viable CD3+CD4+cells that bound the HLA-DR1/HA305−320tetramer were sorted by flow cytometry, and a molecular analysis of expressedTRBgene rearrangements was conducted as described in the Methods. (a) Gating strategy used to identify viable CD3+CD4+tetramer-positive events in: (b) line Flu1, (c) line Flu2 and (d) line Flu3. The flow cytometric gating strategy used to sort these antigen-specific CD4 + T-cell populations is shown in Figure 3a . As shown in Figure 3b–d , expansions of greater magnitude were observed in response to Flu3 (28.7% of CD3 + T cells) compared with either Flu1 or Flu2 (19.4% and 22.6% of CD3 + T cells, respectively). The quantitative clonotypic composition of each tetramer-positive CD4 + T-cell population is shown in Table 1 . The antigen-specific repertoires were markedly oligoclonal and highly skewed in all cases, especially in the Flu3-specific CD4 + T-cell population ( Table 1 ). Furthermore, despite the occurrence of common sequences in the Flu1-, Flu2- and Flu3-specific lines, distinct clonotypes emerged and often predominated. A repeat experiment with the same donor demonstrated a strikingly similar clonotypic composition in response to Flu1, Flu2 and Flu3 peptides with no significant difference (Chi square 0.72; P =0.70) between experiments (data not shown). Furthermore, good concordance was observed with respect to the TRBV profiles obtained by spectratyping for Flu1-specific and Flu2-specific lines ( Fig. 2 ). Thus, C-terminally modified peptides can induce biased clonotypic selection from a common starting pool. Figure 3: Flow cytometric sorting of CD4 + T-cell lines. Short-term T-cell lines were generated from peripheral blood stimulated with the indicated peptides. Viable CD3 + CD4 + cells that bound the HLA-DR1/HA 305−320 tetramer were sorted by flow cytometry, and a molecular analysis of expressed TRB gene rearrangements was conducted as described in the Methods. ( a ) Gating strategy used to identify viable CD3 + CD4 + tetramer-positive events in: ( b ) line Flu1, ( c ) line Flu2 and ( d ) line Flu3. Full size image Table 1 Clonotypic composition of CD4 + T cells expanded using different Flu antigens. Full size table These data show that repertoire composition is altered relative to wild type when basic tail peptides are used to stimulate memory CD4 + T-cell responses ( Figs 2 and 3 , and Table 1 ). This biased selection process suggests that basic residues in the C-terminal tail might preferentially enhance recognition by certain clonotypes, presumably as a function of TCR structure. Improved TCR binding affinity to C-terminally modified peptides The mechanism that drives enhanced recognition of C-terminally modified peptides and the associated repertoire skewing remains unclear, although there is some evidence that length modulation of the C-terminal peptide-flanking region can directly affect T-cell recognition [14] , [28] , [29] . To provide an experimental explanation for this observation, we generated soluble αβ TCRs specific for the HA 305−320 epitope presented by HLA-DR1 (F11 and HA-C6 TCRs), or by either HLA-DR1 or HLA-DR4 (HA1.7 TCR). We also manufactured soluble versions of HLA-DRα1*0101/DRβ1*0101 and HLA-DRα1*0101/DRβ1*0401 bound to Flu1 (HA 305−320 ), Flu2 and Flu3 peptides. Biophysical analysis, using SPR, revealed that the binding affinity of the HA1.7, F11 and HA-C6 TCRs was increased by ∼ 1.4–1.8-fold with Arg substituted into the C-terminus of the peptide-flanking region at P10 (PKYVKQNTLKL R T) and ∼ >2 fold with Arg at P11 (PKYVKQNTLKLA R ) ( Fig. 4 ; Supplementary Fig. S2 ). These data provide the first demonstration that changes in the C-terminal flanking region of MHC-II epitopes can substantially enhance TCR binding affinity, and indicate a mechanism through which peptide flanking residues could influence repertoire selection. Although these increases in TCR/pMHC binding affinity may appear small, we and others have previously reported that even minimal changes in affinity can have a substantial impact on T-cell activation [25] , [30] . Furthermore, these increases in affinity can enhance the avidity of tetramer binding by up to three orders of magnitude (D.K.C and A.G., unpublished observations). 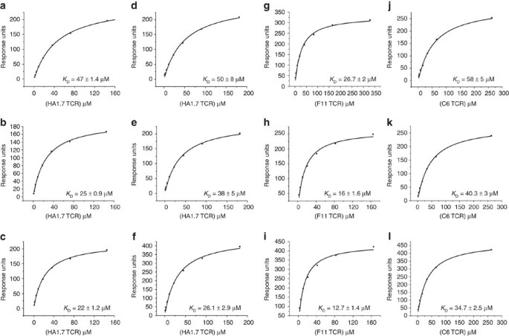Figure 4: The impact of altered C-terminal peptide flanking residues on TCR/pMHC-II affinity. SPR was used to quantify equilibrium binding of the HA1.7, F11 and HA-C6 TCRs to native and altered Flu peptides complexed with HLA-DR1 and HLA-DR4. Representative data from three independent experiments are shown. (a) HA1.7 TCR binding to HLA-DR4 complexed with Flu1 (PKYVKQNTLKLAT). (b) HA1.7 TCR binding to HLA-DR4 complexed with Flu2 (PKYVKQNTLKLRT). (c) HA1.7 TCR binding to HLA-DR4 complexed with Flu3 (PKYVKQNTLKLAR). (d) HA1.7 TCR binding to HLA-DR1 complexed with Flu1. (e) HA1.7 TCR binding to HLA-DR1 complexed with Flu2. (f) HA1.7 TCR binding to HLA-DR1 complexed with Flu3. (g) F11 TCR binding to HLA-DR1 complexed with Flu1. (h) F11 TCR binding to HLA-DR1 complexed with Flu2. (i) F11 TCR binding to HLA-DR1 complexed with Flu3. (j) HA-C6 TCR binding to HLA-DR1 complexed with Flu1. (k) HA-C6 TCR binding to HLA-DR1 complexed with Flu2. (l) HA-C6 TCR binding to HLA-DR1 complexed with Flu3. These data show that modifications in the C-terminal flanking region of peptide antigens restricted by MHC-II can impinge directly on TCR binding, with changes at P11 having greater effects than changes at P10. Substitution to arginine at P10 or P11 markedly increased TCR/pMHC-II binding affinity. Figure 4: The impact of altered C-terminal peptide flanking residues on TCR/pMHC-II affinity. SPR was used to quantify equilibrium binding of the HA1.7, F11 and HA-C6 TCRs to native and altered Flu peptides complexed with HLA-DR1 and HLA-DR4. Representative data from three independent experiments are shown. ( a ) HA1.7 TCR binding to HLA-DR4 complexed with Flu1 (PKYVKQNTLKLAT). ( b ) HA1.7 TCR binding to HLA-DR4 complexed with Flu2 (PKYVKQNTLKL R T). ( c ) HA1.7 TCR binding to HLA-DR4 complexed with Flu3 (PKYVKQNTLKLA R ). ( d ) HA1.7 TCR binding to HLA-DR1 complexed with Flu1. ( e ) HA1.7 TCR binding to HLA-DR1 complexed with Flu2. ( f ) HA1.7 TCR binding to HLA-DR1 complexed with Flu3. ( g ) F11 TCR binding to HLA-DR1 complexed with Flu1. ( h ) F11 TCR binding to HLA-DR1 complexed with Flu2. ( i ) F11 TCR binding to HLA-DR1 complexed with Flu3. ( j ) HA-C6 TCR binding to HLA-DR1 complexed with Flu1. ( k ) HA-C6 TCR binding to HLA-DR1 complexed with Flu2. ( l ) HA-C6 TCR binding to HLA-DR1 complexed with Flu3. These data show that modifications in the C-terminal flanking region of peptide antigens restricted by MHC-II can impinge directly on TCR binding, with changes at P11 having greater effects than changes at P10. Substitution to arginine at P10 or P11 markedly increased TCR/pMHC-II binding affinity. Full size image Interestingly, the previously published ternary structure of the HA1.7 TCR bound to HLA-DR1/HA 305−320 (ref. 31 ) revealed that that the TCR cannot make direct contacts with the short side chains of either Ala at P10 or Thr at P11 in the native Flu1 peptide. Indeed, the closest proximity between the TCR and either P10 or P11 is over 8 Å, which is beyond the limits for atomic contacts ( Fig. 5a ). However, substitution with Arg, which has a long basic side chain, at either P10 or P11 could close this gap and allow further interactions to form between the peptide and the TCR. To investigate this possibility from a theoretical perspective, we modelled the Arg at P10 and Arg at P11 substitutions, using the original structure of the HA1.7 TCR bound to HLA-DR1/HA 305−320 (ref. 31 ) (PDB Code 1FYT) as a guide. This analysis indicated that Arg at either P10 ( Fig. 5b ) or P11 ( Fig. 5c ) could form a salt bridge with Asp28 in the TCR β-chain. These extra bonds could enhance TCR-binding affinity to pMHC-II, and explain the observed differences in both T-cell activation and repertoire selection between the native Flu1 peptide and the basic tail peptides Flu2 and Flu3. Thus, the presence of an Arg in the C-terminal flanking region appears to enhance T-cell activation by increasing the affinity of the TCR/pMHC-II interaction by potentially generating new contacts between the TCR and peptide. 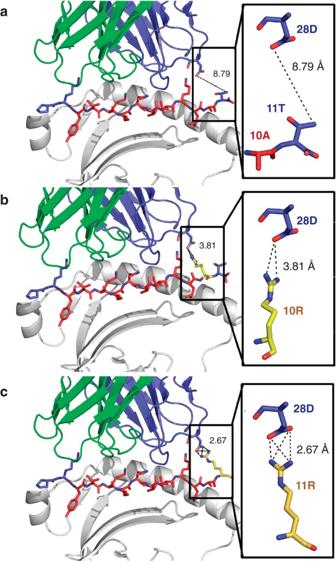Figure 5: Molecular modeling of Arg substitutions in the C-terminal flanking region of the native Flu1 peptide. (a) HA1.7 TCR (TCRα green, TCRβ blue cartoon) bound to HLA-DR1 (grey cartoon) complexed with Flu1 (PKYVKQNTLKLAT; core region red sticks, flanking regions blue sticks). The HA1.7 TCR β-chain is beyond the limits for atomic contacts with either P10 or P11 in the native structure. (b,c) Modelling shows that a new interaction, possibly a salt bridge, could be formed between the HA1.7 TCR β-chain residue Asp28 and Arg substituted at either position 10 (b) or 11 (c) of the HA peptide. This new interaction could explain the increase in affinity observed for cognate TCR binding to Flu2 and Flu3 compared with Flu 1. Figure 5: Molecular modeling of Arg substitutions in the C-terminal flanking region of the native Flu1 peptide. ( a ) HA1.7 TCR (TCRα green, TCRβ blue cartoon) bound to HLA-DR1 (grey cartoon) complexed with Flu1 (PKYVKQNTLKLAT; core region red sticks, flanking regions blue sticks). The HA1.7 TCR β-chain is beyond the limits for atomic contacts with either P10 or P11 in the native structure. ( b , c ) Modelling shows that a new interaction, possibly a salt bridge, could be formed between the HA1.7 TCR β-chain residue Asp28 and Arg substituted at either position 10 ( b ) or 11 ( c ) of the HA peptide. This new interaction could explain the increase in affinity observed for cognate TCR binding to Flu2 and Flu3 compared with Flu 1. Full size image MHC-II molecules present peptide epitopes that include flanking regions, that can extend beyond the MHC-II binding groove, to CD4 + T cells. Structural studies have demonstrated that cognate TCRs primarily engage amino acids in the core nonamer region of the epitope situated within the MHC-II groove, although some contacts can also be made with residues in the flanking regions [31] , [32] . Perhaps surprisingly, it appears that these flanking residues can influence CD4 + T-cell recognition [10] , [29] . Indeed, we have shown previously that non-bound C-terminal flanking residues can alter T-cell activation in an MHC allele-transcending fashion; these effects apply to T-cell clones, lines and polyclonal populations directly ex vivo [11] . However, the mechanism for this potentially important phenomenon, and the means by which it could influence TCR selection and activation, is currently unknown. Several hypotheses have been put forward to explain how substitutions in the residues that flank the core of an antigenic peptide might influence T-cell responses. These include altered peptide binding to the restricting HLA element, effects on cellular uptake and antigen processing and; changes in pMHC-II conformation [33] . To explore the role of MHC-II peptide-flanking regions, we screened hemaggluttinin-specific CD4 + T-cell clones using families of peptides, each with a range of different amino-acid substitutions in the C-terminus flank at P10 or P11, and confirmed that basic residues were among the most favoured. The observation that substitution of either the P10 Ala or P11 Thr of the universal HA 305−320 epitope with an Arg residue resulted in altered recognition by cognate CD4 + T cells provided a good model system to examine the role of the C-terminal flanking region in more detail. In a previous study, we excluded the possibility that these 'basic tail' peptides exhibit improved binding to the restricting MHC element in this system [11] . We therefore proceeded to examine whether such substitutions could influence binding to cognate TCRs. Using SPR, we found that the presence of an Arg at P10 or P11 in the C-terminal epitope flanking region enhanced TCR/pMHC-II affinity. This enhanced binding provided a molecular mechanism for the observed alterations in the immunogenicity of basic tail peptides. However, such improved binding affinity was also surprising, considering that the previously published ternary structure of the HA1.7 TCR bound to HLA-DR1/HA 305−320 (ref. 31 ) revealed that the TCR does not make direct contacts with the short side chains of either Ala at P10 or Thr at P11 in the native Flu1 peptide. Molecular modelling suggested that substitution at P10 or P11 with Arg, which has a long basic side chain, could close this gap and allow further interactions to form between the peptide and the TCR. These extra bonds could enhance the binding affinity between the TCR and peptide, and could explain the differences in T-cell activation and repertoire selection between the native Flu1 peptide and the basic tail peptides Flu2 and Flu3. Thus, the introduction of a positively charged, longer amino-acid side chain in the C-terminal flanking region could allow for the formation of new bonds between the TCR and peptide, although formal proof that such bonds exist awaits further structural characterization. Regardless, the presence of an Arg in the C-terminal flanking region seemed to enhance T-cell activation by increasing the affinity of TCR for pMHC-II. Intriguingly, when basic tail peptides were used to stimulate memory T-cell responses, striking differences were observed in repertoire composition despite similar numerical expansions. This biased selection process suggests that basic residues in the C-terminal tail might preferentially enhance recognition by certain clonotypes, presumably as a function of TCR structure. Further studies are ongoing to explore the underlying basis for these differential effects. In summary, we have shown that basic tail peptides can enhance TCR/pMHC-II affinities into the range typically observed for TCR/pMHC-I interactions [18] . This exciting observation suggests that universal augmentation of pMHC-II antigens through particular C-terminal modifications may be a realistic option, with attendant implications for vaccination and other immune system interventions. Peptides Peptides were synthesized commercially to >80% purity (EMC Microcollections, Tubingen, Germany). The following peptides were used: the universal influenza epitope HA 305−320 (Flu1), PKYVKQNTLKLAT; C-terminally modified variants with Arg at P10 or P11 (Flu2=PKYVKQNTLKLRT, Flu3=PKYVKQNTLKLAR); and a peptide library synthesized with variant peptides containing substitutions of the native amino acids in the C-terminal flanking region at P10 and P11. The substitutions in each library peptide were Gly, Arg, Lys, Glu, Ser, Asp, Leu, Val, Phe and Tyr, covering conservative, basic, acidic, aliphatic and bulky hydrophobic changes. Cell culture Epstein–Barr virus-immortalized B-cell lines (BCLs) were cultured in RPMI (Invitrogen) supplemented with 10% fetal calf serum (FCS; Invitrogen), 2 mM glutamine, 100 μg ml −1 streptomycin, 100 IU ml −1 penicillin and 25 mM HEPES (Sigma) (RPMI–FCS medium). All T-cell lines and clones were cultured in RPMI supplemented with 7% human AB serum, 2 mM glutamine, 100 μg ml −1 streptomycin, 100 IU ml −1 penicillin and 25 mM HEPES (RPMI–AB medium). PBMCs were obtained from two HLA-DR1 + donors by density gradient centrifugation of heparinized blood layered onto an equal volume of Lymphoprep (Axis-Shield). All human samples were used in accordance with UK guidelines. T-cell lines and clones were generated as described previously [11] , [34] . Antigen-specific T cells were cloned out either using HLA-DR1/HA 305−320 tetramer staining and cell sorting, or by limiting dilution assays. Three clones specific for HLA-DR1/HA 305−320 (HA-C6, HA-C5 and HA-CA) were used to screen peptide variants; a further clone (F11) was used for biophysical work. Clonality was confirmed by sequencing TRA and TRB gene rearrangements; HLA restriction was confirmed by using peptide titrations in the presence of HLA-DR1 + matched and mismatched BCLs, together with another clone (HA1.7) restricted by HLA-DR1 and HLA-DR4 (ref. 35 ). Screening T-cell clones The frequency of specific IFN-γ producing T cells was measured by ELISpot assay as described previously [10] . Briefly, mouse anti-human IFN-γ antibody 1-DIK (Mabtech) was added to a polymer-backed 96-well filtration ELISpot plate (MAIP-S-4510; Millipore). Plates were washed thoroughly and blocked with 100 μl of 10% FCS. Duplicate wells were set up with 200 T cells and 1,500 BCLs (HLA-DR1 homozygous) per well with 0.1–1 μg ml −1 of peptide. The plate was incubated at 37 °C for 16–18 h, then developed according to standard protocols. Wells were considered positive if the number of spots was at least twice that observed in the control (no antigen) wells and >5 spots per well. T-cell proliferation was measured by incorporation of 3[H] thymidine (Amersham Life Science). Spectratyping PBMCs were isolated from healthy HLA-DR1 + donors and short-term lines specific for Flu1 and Flu2 were set up over a period of 8–10 days. Cells were then stained with PE-conjugated HLA-DR1/HA 305−320 tetramer (2 μg ml −1 ) for 24 min at 37 °C, followed by 2 μl αCD4-FITC (Miltenyi) for 20 min at 4 °C. Tetramer-labelled cells were then either enriched using anti-PE MACS beads (Miltenyi) according to the manufacturer's instructions or isolated using a MoFlo cell sorter (BD Biosciences). Purity was assessed by flow cytometry. Typically, 1–2×10 4 antigen-specific T cells were obtained. Both the tetramer-positive and tetramer-negative fractions were processed, together with negative controls comprising unstimulated PBMCs. Determination of TRBV gene usage and immunoscope analysis was performed as described previously [36] . Briefly, total RNA was extracted using the RNeasy mini-kit (Qiagen) according to the manufacturer's specifications. cDNA was then prepared by RNA reverse-transcription with 0.5 μg μl −1 oligo (dT)17 and 200 U of Superscript II reverse transcriptase (Invitrogen). An aliquot of the cDNA synthesis reaction was amplified with each of 24 TRBV family-specific primers as previously described [37] , together with a TRBC primer and a minor groove binder TaqMan probe (Applied Biosystems). Real-time quantitative PCR was carried out using an ABI 7300 device (Applied Biosystems). Subsequently, 2 μl of each amplification reaction was used as template in run-off reactions with a nested fluorescent TRBC-specific primer. In these reactions, all PCR products were copied into fluorescently-labelled single-stranded DNA fragments, irrespective of their TRBJ gene usage or CDR3β sequence. These fluorescent products were separated on an ABI-PRISM 3730 DNA analyzer (Applied Biosystems). The size and intensity of each band were analysed with Immunoscope software [4] , [36] . Fluorescence intensity was plotted in arbitrary units on the y axis, with the x axis corresponding to CDR3β length in amino acids. TCR clonotyping Cell lines specific for HLA-DR1/HA 305−320 were stained first with 1 μl, diluted 1:40, LIVE/DEAD Fixable Violet Dead Cell Stain (Invitrogen/Life Technologies) for 15 min at room temperature in the dark, then with allophycocyanin-conjugated tetramer for 20 min at 37 °C. Subsequently, cells were stained for 20 min at room temperature in the dark with the following monoclonal antibodies: 3 μl αCD3-FITC and 2 μl αCD8-PECy7 (BD Pharmingen); and 0.2 μl αCD4-PECy5.5, αCD14-Pacific Blue and αCD19-Pacific Blue (Caltag/Life Technologies). Tetramer-labelled CD3 + CD4 + cells were sorted viably at >98% purity using a customized 20-parameter FACSAria II flow cytometer (BD Biosciences) directly into 1.5 ml microtubes containing 100 μl RNAlater (Applied Biosystems). Clonotypic analysis was then conducted using a template-switch anchored reverse-transcription PCR to amplify all expressed TRB gene products without bias using a template-switch anchored reverse transcription PCR with a 3′-TRB constant region primer (5′-GGCTCAAACAAGGAGACCT-3′), as described previously with minor modifications [38] , [39] . Amplicons were subcloned, sampled, sequenced and analysed as described previously [39] , [40] . The international ImMunoGeneTics nomenclature [41] is used to display all TCR sequence data. Generation of expression plasmids The HA1.7, F11 and HA-C6 TCRs were generated from the corresponding CD4 + T-cell clones as described previously [42] . All sequences were confirmed by automated DNA sequencing (Lark Technologies). A disulphide-linked construct was used to produce the soluble domains (variable and constant) for both the TCRα and TCRβ chains [43] . The HLA-DRα*0101 chain, tagged with a biotinylation sequence, DRβ*0101 chain and DRβ*0401 chain were also cloned and used to produce the pMHC-II molecules [18] . All constructs were inserted into separate pGMT7 expression plasmids under the control of the T7 promoter. Protein expression and purification Competent Rosetta DE3 Escherichia coli cells were used to produce the HA1.7, F11 and HA-C6 TCRα and TCRβ chains, the HLA-DRα1*0101 chain, the DRβ1*0101 chain and the DRβ1*0401 chain in the form of inclusion bodies using 0.5 mM isopropyl-β-d-thiogalactoside to induce expression as described previously [42] . The HLA-DRα1*0101 chain, the DRβ1*0101 chain and the DRβ1*0401 chain were purified into 8 M urea buffer (8 M urea, 20 mM TRIS pH8.1, 0.5 mM EDTA, 30 mM DTT) by ion exchange using a Poros50HQ column (GE Healthcare) to remove bacterial impurities. For a 1-litre TCR refold, 30 mg of TCRα chain was incubated for 15 min at 37 °C with 10 mM dithiothreitol (DTT) and added to cold refold buffer (50 mM TRIS pH8.1, 2 mM EDTA, 2.5 M urea, 6 mM cysteamine hydrochloride and 4 mM cystamine). After 15 min, 30 mg of TCRβ chain, also incubated for 15 min at 37 °C with 10 mM DTT, was added. For a 1-litre pMHC-II refold, 2 mg of HLA-DRα1*0101 chain was mixed with 2 mg of either the HLA-DRβ1*0101 chain or the DRβ1*0401 chain and 0.5 mg of peptide for 15 min at 37 °C with 10 mM DTT [44] . The following peptides (generated by Peptide Protein Research) were used in separate refolds: PKYVKQNTLKLAT, PKYVKQNTLKL R T and PKYVKQNTLKLA R (basic tail peptide-flanking region changes are denoted in bold). This mixture was then added dropwise to cold refold buffer (25% glycerol, 20 mM TRIS pH8.1, 1 mM EDTA, 2 mM glutathione reduced, 0.2 mM glutathione oxidized). Refolds were incubated for 72 h at 4 °C. Dialysis was carried out against 10 mM TRIS pH 8.1 until the conductivity of the refolds was <2 mS cm −1 . The refolds were then filtered, ready for purification steps. Refolded proteins were purified initially by ion exchange using a Poros50HQ column (GE Healthcare) and then gel-filtered into BIAcore buffer (10 mM HEPES pH 7.4, 150 mM NaCl, 3 mM EDTA and 0.05% (v/v) Surfactant P20) using a Superdex200HR column (GE Healthcare). Protein quality was analysed by Coomassie-stained SDS–PAGE. Biotinylated pMHC-II was prepared as described previously [45] . Surface plasmon resonance analysis Binding analysis was performed using a BIAcore 3000 and a BIAcore T100 (GE Healthcare) equipped with a CM5 sensor chip, as reported previously [42] , [46] . Between 200 and 400 response units of biotinylated pMHC-II was immobilized on streptavidin, which was chemically linked to the chip surface; pMHC-II was injected at a slow-flow rate (10 μl min −1 ) to ensure uniform distribution on the chip surface. The HA1.7, F11 and HA-C6 TCRs were purified and concentrated to ∼ 100 μM on the day of SPR analysis to minimize TCR aggregation. For equilibrium analysis, eight serial dilutions were carefully prepared in triplicate for each sample and injected over the relevant sensor chip at a flow rate of 45 μl min −1 at 25 °C. Results were analysed using BIAevaluation 3.1, Microsoft Excel and Origin 6.1. The equilibrium binding constant ( K D ) values were calculated using a nonlinear curve fit ( y =(P 1 x )/(P 2 + x )). How to cite this article: Cole, D. K. et al . Modification of the carboxy-terminal flanking region of a universal influenza epitope alters CD4 + T-cell repertoire selection. Nat. Commun. 3:665 doi: 10.1038/ncomms1665 (2012).